The isotopic effects of deuteration on optoelectronic properties of conducting polymers The attractive optoelectronic properties of conducting polymers depend sensitively upon intra- and inter-polymer chain interactions, and therefore new methods to manipulate these interactions are continually being pursued. Here, we report a study of the isotopic effects of deuterium substitution on the structure, morphology and optoelectronic properties of regioregular poly(3-hexylthiophene)s with an approach that combines the synthesis of deuterated materials, optoelectronic properties measurements, theoretical simulation and neutron scattering. Selective substitutions of deuterium on the backbone or side-chains of poly(3-hexylthiophene)s result in distinct optoelectronic responses in poly(3-hexylthiophene)/[6,6]-phenyl-C61-butyric acid methyl ester (PCBM) photovoltaics. Specifically, the weak non-covalent intermolecular interactions induced by the main-chain deuteration are shown to change the film crystallinity and morphology of the active layer, consequently reducing the short-circuit current. However, side-chain deuteration does not significantly modify the film morphology but causes a decreased electronic coupling, the formation of a charge transfer state, and increased electron–phonon coupling, leading to a remarkable reduction in the open circuit voltage. The optoelectronic properties of conjugated polymers are known to depend sensitively upon intra- and inter-polymer chain interactions coupled to molecular vibration modes. Thus, new methods to manipulate and control these interactions are continually being pursued. Experimental and theoretical studies have already shown that isotope effects have a significant influence on the thermal, elastic and vibrational properties of materials, due to their different atomic masses, volume, and spin [1] . More specifically, several recent studies have provided evidence for significant deuterium isotope effects on the electroluminescence and magnetic responses in organic semiconductors. For example, Hwang and Tong [2] reported that deuteration of the small molecule aluminium tris(8-hydroxyquinoline) (Alq 3 ) can significantly improve the light emitting efficiency and high voltage stability in organic light emitting diodes. Similarly, Nguyen et al. [3] found that deuteration of a polyphenylenevinylene-based conjugated polymer can effectively change the hyperfine interaction in organic materials, thereby influencing spin transport, magnetoconductance and magnetoelectroluminescence in organic spin valve and organic light-emitting diode (OLED) devices. Deuterium substitution has also been shown to change the superconducting transition temperature ( T c ) in organic superconductors due to a reduced lattice volume and internal pressure originating from the smaller zero-point spacing of the C-D bonds [4] . Despite these interesting observations, to date there has not been any fundamental discussion about how isotopic substitution alters the optoelectronic properties of conducting polymers. This is likely due to the common belief that deuteration does not appreciably change the chemical and optoelectronic properties of compounds because compounds incorporating different isotopes generally exhibit nearly identical electronic structure. This assumption, however, neglects the importance of non-covalent π - π interactions in conducting polymers that are especially important for their optoelectronic properties. Due to the large relative mass difference of deuterium and hydrogen, the physical properties such as polarity, polarizability and molecular volume of the protonated and deuterated polymers could be different. These factors could in principle lead to a change of non-covalent (for example, hydrogen bonding, CH- π , π - π , and cation- π ) interactions upon deuteration. There have been a few studies in the past showing that deuteration of C-H oscillators can lead to decreased non-covalent interactions in a non-conjugated system, but the observed differences were too small to be statistically significant, and the exact causality could therefore not be established unambiguously [5] , [6] , [7] , [8] . It should also be noted that isotopic substitution in conducting polymers is a widely used technique to increase the scattering length density (SLD) contrast of polymers in neutron scattering measurements [6] , [7] , [8] . This is due to an increasing interest in taking advantage of the nanometer scale resolution provided by neutron reflectometry (NR)/scattering to probe the structure, interface and morphology of bulk heterojunctions (BHJ) in organic photovoltaics (OPV) [9] , [10] , [11] , [12] , [13] , [14] , [15] to determine not only the nanoscopic heterogeneity of donor/acceptor components, but their degree of mixing and the vertical composition. The nanoscopic morphological information provided by isotopic substitution is highly relevant to understand exciton diffusion and charge transport in these devices [9] , [10] , [11] , [12] , [13] , [14] , [15] ; however, deuteration is commonly believed to have little effect on morphology. Only recently, small-angle neutron scattering revealed that deuterium substitution can significantly influence the phase separation kinetics and morphology in some polymer blend systems [16] , [17] . Little work on the potential effects of deuterium substitution in the phase behaviour of conducting polymers and the interpretation of corresponding neutron measurements has been performed, and is urgently needed. In this paper, we develop a series of regioregular poly(3-hexylthiophene) (rr-P3HT) isotopes by selectively substituting deuterium on its backbone (main-chain deuteration, MD-P3HT) or alkyl group (side-chain deuteration, SD-P3HT). We find that selective deuteration contributes remarkably to the optoelectronic properties of conductive P3HT polymers in OPVs. Furthermore, we systematically investigate the effects of deuteration on different photovoltaic processes, and have correspondingly understood the structure–performance relationship by combining multiple optical and structure analysis techniques. Materials characterization and device performance P3HT is a typical semiconducting polymer used in organic electronics that has been studied intensely [18] , [19] . Moreover, P3HT/PCBM is an excellent system to elucidate the isotope effect in deuterated polymers because P3HT and PCBM naturally exhibit a large contrast in neutron SLD, making the detection of potential structural changes more probable. To make these measurements possible, three P3HT polymers are synthesized, two partially deuterated and one protonated. The partially deuterated P3HT polymers are selectively deuterated on the thiophene ring (MD-P3HT) or the alkyl side-chain position (SD-P3HT) as shown in Fig. 1a . The detailed synthesis processes are described in the Methods Section and Supplementary Fig. 1 . Considering that molecular weight and regioregularity of P3HT can impact the molecular packing and device performance [19] , [20] , [21] , great care is taken to ensure that all polymers have similar values for average molecular weight ( M w ), regioregularity (rr) and polydispersity index (PDI). The M w , rr and PDI are 14 kg mol −1 , 98.7% and 1.15 for the protonated P3HT; 11.2 kg mol −1 , 98.3% and 1.21 for the MD-P3HT; and 14 kg mol −1 , 98.6% and 1.17 for the SD-P3HT. Several studies have previously demonstrated that P3HT molecular weight variations in the range of 10–20 kg mol −1 do not significantly affect the morphology and device performance of the pristine polymer or P3HT/PCBM-based photovoltaics [22] , [23] , [24] . In addition, the Ni residues in the highly pure protonated and deuterated P3HT polymers synthesized for this study were measured by inductively coupled plasma mass spectroscopy to be less than 0.0014, wt.%, which is 50 times smaller than the threshold concentration of metal impurities for noticeable effects on device performance in previous studies [25] , [26] , [27] . Therefore, we exclude the impact of the molecular weight difference and metal residues on the measured optoelectronic properties between the deuterated and protonated P3HT polymers in this work. 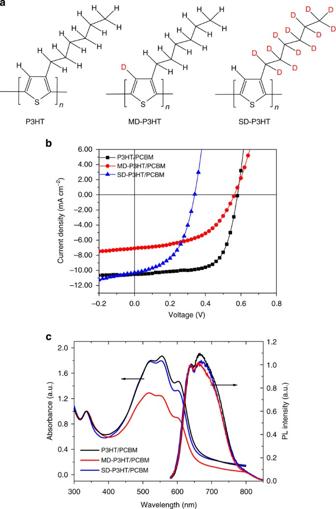Figure 1: Device performance and optical properties. (a) Chemical structure of P3HT, MD-P3HT and SD-P3HT (b) Typical J-V characteristics of the three P3HT isotopes blended with PCBM. (c) UV–vis absorption (normalized to the absorption peak of PCBM) and photoluminescence spectra of P3HT isotopes mixed with PCBM after thermal annealing. Figure 1b compares the current density ( J ) versus voltage ( V ) curves of deuterated and protonated P3HT/PCBM photovoltaic devices, and the important device performance parameters are summarized in Table 1 . They include short-circuit current ( I sc ), open circuit voltage ( V oc ), fill factor (FF) and power conversion efficiency (PCE). After the main-chain deuteration of P3HT, the PCE drops by a half from 4.0% to 2.0% due to both a reduced I sc of 7.0 mA cm −2 and a FF of 51.2%. Similarly, the deuteration of the alkyl side chain also results in a reduced PCE of 1.8%. Interestingly, the major efficiency loss of SD-P3HT/PCBM originates from a significantly reduced V oc of 0.24 V and a FF of 50.3%, whereas an almost unchanged I sc is maintained. Figure 1c shows the UV–vis absorption and photoluminescence (PL) spectra of deuterated P3HT/PCBM blend films. All P3HT isotopes exhibit three absorption peaks centred at 515 and 550 nm arising from 0–0 and 0–1 intrachain excitation, respectively, and at 600 nm associated with π - π interchain interactions [28] . In addition, all exhibit the same absorption edge at 650 nm and a photoluminescence peak at 665 nm. Figure 1: Device performance and optical properties. ( a ) Chemical structure of P3HT, MD-P3HT and SD-P3HT ( b ) Typical J-V characteristics of the three P3HT isotopes blended with PCBM. ( c ) UV–vis absorption (normalized to the absorption peak of PCBM) and photoluminescence spectra of P3HT isotopes mixed with PCBM after thermal annealing. Full size image Table 1 Device performances of three P3HT isotopes. Full size table Raman spectroscopy As hydrogen is substituted with deuterium, the change in the vibrational modes of P3HT can be directly revealed by Raman spectroscopy. 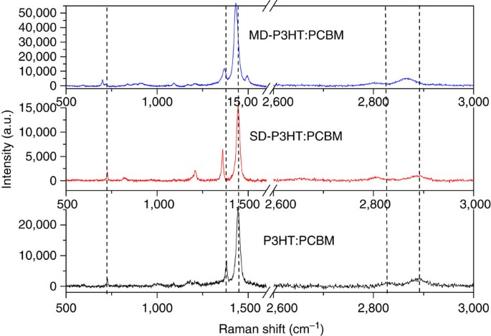Figure 2: Raman spectra. Raman spectroscopy measurements of different P3HT isotopes mixed with PCBM reveal the change in vibrational modes of P3HT. Figure 2 and Table 2 present Raman spectroscopy measurements of different P3HT isotopes mixed with PCBM. Upon side-chain deuteration, the C-C in-plane ring skeleton modes at 1,380 cm −1 and the C-H symmetric stretching mode at 2,822 cm −1 are shifted downwards by almost 20 cm −1 because the heavier deuterium decreases the vibrational frequency [29] . The Raman shift of the C-H stretching mode is in agreement with the expected isotope shift based on the square root of the C-D/C-H mass ratio [3] , and the vibrational frequency of the C-S-C ring in-plane skeleton mode at 728 cm −1 remains unchanged, suggesting that the vibrational modes of the thiophene backbone are not affected by side-chain deuteration. In contrast, after deuteration of the thiophene backbone, the in-plane vibrational C-S-C mode and C-H stretching mode blue-shift to 702 and 2,788 cm −1 , respectively, suggesting that backbone deuteration is more effective than side-chain deuteration in affecting the vibrational modes of the thiophene backbone. This leads to changes in the intermolecular interaction of the P3HT, and is consistent with the features observed in the UV–vis and PL measurements. The significant Raman shifts also indicate that we were successful in selectively deuterating P3HT on both the thiophene backbone and alkyl side chain position. As shown in Supplementary Fig. 2 , the singlet’s emission lifetimes in MD-P3HT and SD-P3HT blend films are significantly reduced when compared with that of the P3HT blend film, suggesting that deuteration affects excited state dynamics and the subsequent electron transfer from the excited P3HT to the PCBM acceptor. Figure 2: Raman spectra. Raman spectroscopy measurements of different P3HT isotopes mixed with PCBM reveal the change in vibrational modes of P3HT. Full size image Table 2 Raman shift of three P3HT isotopes when blending with PCBM. Full size table Morphology characterization The photoactive layer morphology is important to the charge separation and transport processes, which are critical for OPV performance [30] , [31] . We examine whether deuterium substitution will affect film structure, crystallinity and morphology. In Fig. 3a , atomic force microscope phase images clearly show the characteristic nanofibrillar structures in both P3HT/PCBM and SD-P3HT/PCBM films, suggesting the formation of highly crystalline P3HT domains in blend films [21] . The average size of the nanofibrils is ~20±3 nm, which is consistent with the desirable morphology [32] . In contrast, there is no clear indication of P3HT crystalline fibrils in the MD-P3HT/PCBM film, which may indicate that MD-P3HT is less crystalline or perhaps amorphous. To obtain better insight into the morphology of the film, we also carried out energy-filtered transmission electron microscopy as shown in Fig. 3b . Note that the energy window is centred at 19±4 eV to provide maximum contrast for P3HT, and as a result, the bright regions in the micrographs correspond to P3HT-rich domains [33] . It was observed that the P3HT and SD-P3HT domains overlap with each other over the whole film, indicating the formation of an interpenetrating network with no visible isolated P3HT fibrils. In contrast, the MD-P3HT/PCBM exhibits poor connectivity and a larger average domain size of 29 nm. Consequently, the interfacial area between the polymer and PCBM is reduced, hindering charge separation and charge transport in the percolating networks, ultimately leading to a lowered I sc and FF. Selected area diffraction was also performed, and the insets of Fig. 3b show the patterns. Two diffraction rings, corresponding to the (010) reflection of P3HT and the PCBM nanocrystallites [32] , respectively, are observed in the P3HT/PCBM and SD-P3HT/PCBM blend films. The MD-P3HT/PCBM film’s diffraction pattern, however, only shows the diffusive ring of PCBM. The absence of the (010) diffraction ring in this case further confirms the low crystallinity of the MD-P3HT crystals. To analyse the material more quantitatively, we plot the residual intensity of the selected area diffraction pattern as a function of the scattering vector, q z , by integrating the diffraction intensity over the electron diffraction ring shown in Fig. 3c . A clear peak appears at 1.6 Å −1 in both the P3HT/PCBM and SD-P3HT/PCBM blends that can be ascribed to the intermolecular π - π stacking distance ( d =0.38 nm) of P3HT. We note the P3HT/PCBM films exhibit a stronger (010) peak intensity when compared with the SD-P3HT/PCBM films, thereby indicating a superior degree of crystallinity and a strong intermolecular interaction. In contrast, the MD-P3HT/PCBM blend film only exhibits a faint shoulder of the (010) peak, indicating that it possesses the weakest intermolecular interaction. Interestingly, it should be noted that the (010) peak position of SD-P3HT shows a slight shift towards larger d spacing when compared with that of P3HT, and should necessarily lead to a decreased overlap between electronic wave functions between adjacent molecules, ultimately resulting in reduced charge carrier mobility. 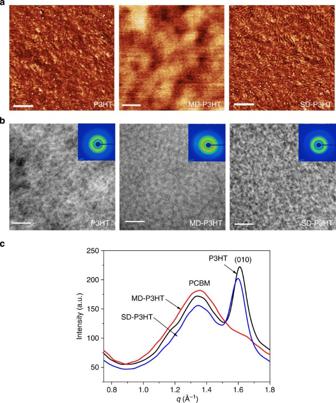Figure 3: Morphology characterizations. (a) AFM phase images of P3HT, MD-P3HT and SD-P3HT blended with PCBM after thermal annealing (scale bar, 200 nm). (b) Energy-filtered TEM images of P3HT, MD-P3HT and SD-P3HT blended with PCBM after thermal annealing (scale bar, 100 nm). Each film is imaged with 19±4 eV, where inelastic scattering is more intense for P3HT. Insets of Fig. 3b show the selected area electron diffraction patterns and (c) corresponding integrated diffraction intensity plots of P3HT, MD-P3HT and SD-P3HT blended with PCBM after thermal annealing. Figure 3: Morphology characterizations. ( a ) AFM phase images of P3HT, MD-P3HT and SD-P3HT blended with PCBM after thermal annealing (scale bar, 200 nm). ( b ) Energy-filtered TEM images of P3HT, MD-P3HT and SD-P3HT blended with PCBM after thermal annealing (scale bar, 100 nm). Each film is imaged with 19±4 eV, where inelastic scattering is more intense for P3HT. Insets of Fig. 3b show the selected area electron diffraction patterns and ( c ) corresponding integrated diffraction intensity plots of P3HT, MD-P3HT and SD-P3HT blended with PCBM after thermal annealing. Full size image Thin film structure and transport characterization The isotope effects of deuteration on the molecular ordering and interchain packing of P3HT in the blend films is further examined with grazing incidence wide-angle and small-angle X-ray scattering (GIWAXS and GISAXS) measurements using a synchrotron X-ray radiation source as shown in Fig. 4 and also in Supplementary Fig. 3 . The GIWAXS profiles from both non-deuterated and deuterated blend films exhibit out-of-plane (l00) and in-plane (010) reflection patterns, [19] indicating a well-organized lamellar structure oriented edge-on with the substrate. MD-P3HT exhibits the lowest crystallinity among the three polymers, as evidenced by the weakest (100) and (010) diffraction intensities. This observation is consistent with the TEM results. The ratio of out-of-plane (100) to in-plane (100) intensities are found to be 239, 32 and 90 for P3HT/PCBM, MD-P3HT/PCBM and SD-P3HT/PCBM film blends, respectively, implying that the population of edge-on crystallites for deuterated P3HT is much less than that for protonated P3HT. Moreover, randomly oriented crystallites will lead to lower carrier mobility, and probably result in a small I sc and worse photovoltaic performance. As shown in Supplementary Fig. 3 and Supplementary Table 1 , the GISAXS results indicate that the R g,1 (54.8~56.2 Å) and R g,2 (95.5~99.7 Å), corresponding to PCBM domains with two significantly different sizes, were essentially identical, which implies that deuteration of P3HT does not significantly affect the size of the PCBM domains in the blend films. The deuteration effect on charge transport is further examined with the OFET configuration shown in Supplementary Fig. 4 . After deuteration, the average mobility is reduced to 3.5 × 10 −3 cm 2 V −1 s −1 (SD-P3HT) and 1.1 × 10 −3 cm 2 V −1 s −1 (MD-P3HT), which is almost one order of magnitude lower than that of protonated P3HT (2.5 × 10 −2 cm 2 V −1 s −1 ). This reduced mobility indicates inefficient charge transport in MD-P3HT/PCBM OPV devices. When combined with the above structural measurements, we are able to conclude that low crystallinity, more random crystallite orientation, and weak π - π intermolecular interaction may be the major reasons for the low short circuit current I sc observed in the MD-P3HT/PCBM BHJ devices. 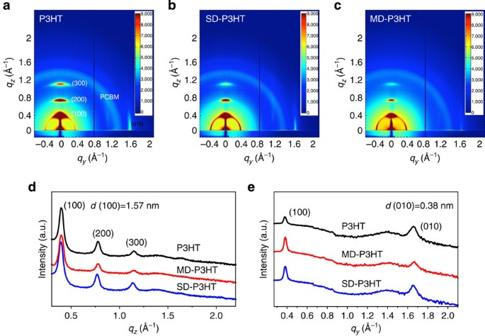Figure 4: Two-dimensional GIWAXS plots (a) P3HT:PCBM, (b) SD-P3HT:PCBM and (c) MD-P3HT:PCBM films annealed at 140 °C. (d) Vertical and (e) horizontal linecuts of the films.qzandqyare the perpendicular and parallel wave vector transfer with respect to substrate surface. Figure 4: Two-dimensional GIWAXS plots ( a ) P3HT:PCBM, ( b ) SD-P3HT:PCBM and ( c ) MD-P3HT:PCBM films annealed at 140 °C. ( d ) Vertical and ( e ) horizontal linecuts of the films. q z and q y are the perpendicular and parallel wave vector transfer with respect to substrate surface. Full size image Electroluminescence In order to understand the origin of reduced V oc observed in the SD-P3HT/PCBM blend, the electroluminescence emission from the protonated and deuterated P3HT/PCBM blend was directly monitored and correlated with V oc . As shown in Fig. 5b , a weak broad infrared emission peaked at 1,210 nm with a shoulder at 1,410 nm in P3HT/PCBM blend are observed. This new emission peak shows a significant red shift compared with the emission from single component P3HT at 660 nm and PCBM emission at 735 nm, and can be attributed to the charge transfer emission formed at the P3HT/PCBM interface [34] . MD-P3HT/PCBM shows the same charge transfer emission without a clear spectral shift, implying the same energy level for the charge transfer state. This result is consistent with the unchanged V oc after the main-chain deuteration. In the SD-P3HT/PCBM device, however, no clear charge transfer emission is observed between 800 and 1800, nm, our detection range. 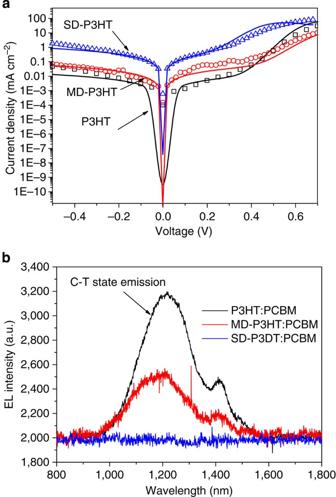Figure 5: The origin of reducedVOC. (a)J-Vcharacteristics in the dark condition for P3HT, MD-P3HT and SD-P3HT based OPVs. Solid lines are fitted to the experimental dark curve using the equivalent circuit model and the parameters inSupplementary Table 2. (b) Electroluminescence spectra from charge-transfer state in P3HT/PCBM, MD-P3HT/PCBM and SD-P3HT/PCBM devices. Figure 5: The origin of reduced V OC . ( a ) J-V characteristics in the dark condition for P3HT, MD-P3HT and SD-P3HT based OPVs. Solid lines are fitted to the experimental dark curve using the equivalent circuit model and the parameters in Supplementary Table 2 . ( b ) Electroluminescence spectra from charge-transfer state in P3HT/PCBM, MD-P3HT/PCBM and SD-P3HT/PCBM devices. Full size image Neutron Reflectometry In order to investigate the effect of deuteration on the vertical phase morphology of P3HT/PCBM blends, we have conducted NR measurements for blend films. 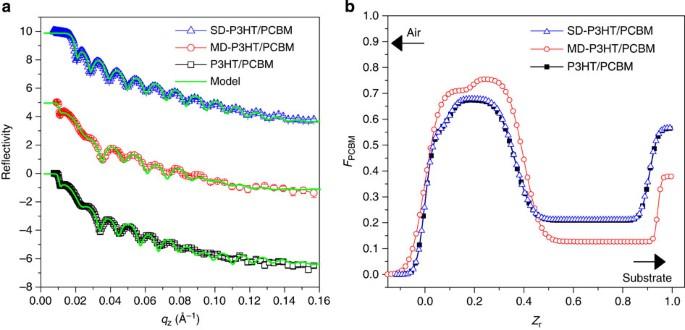Figure 6: Neutron reflectometry. (a) The reflectivity data for P3HT, MD-P3HT and SD-P3HT/PCBM samples. Markers denote the experimental data and the solid lines represent the best fits to the neutron reflectometry data of samples, (b) PCBM volume fraction profiles of the films from which best fits to the experimental data were achieved. The curves for SD-P3HT/PCBM and P3HT/PCBM are overlapped together. Figure 6a shows the neutron reflectivity curves for each blend film. Four-layer models give rise to best fits for all films that are consistent with previously reported results [14] , [35] . The volume fraction profiles of P3HT/PCBM and SD-P3HT/PCBM in Fig. 6b are essentially identical in terms of the vertical phase morphology. The MD-P3HT/PCBM sample shows a similar four-layer pattern; however, the composition profile of the film is clearly different from the films of P3HT/PCBM and SD-P3HT/PCBM. Specifically, more PCBM is accumulated in the surface layer and the mid-layer adjacent to the surface layer in the MD-P3HT/PCBM film. Figure 6: Neutron reflectometry. ( a ) The reflectivity data for P3HT, MD-P3HT and SD-P3HT/PCBM samples. Markers denote the experimental data and the solid lines represent the best fits to the neutron reflectometry data of samples, ( b ) PCBM volume fraction profiles of the films from which best fits to the experimental data were achieved. The curves for SD-P3HT/PCBM and P3HT/PCBM are overlapped together. Full size image As shown in Fig. 1b , clearly the device performance difference resulting from substituting a deuteron for a proton in the thiophene backbone versus an alkyl side chain suggests that main-chain and side-chain deuteration play different roles in optoelectronic processes such as light absorption, charge transfer and transport in BHJ OPV. We note that MD-P3HT/PCBM shows a smaller absorption coefficient and weaker absorption shoulder compared with the P3HT/PCBM and SD-P3HT/PCBM blends. The deuterium isotope effect usually considers only the effects of changes in interactions upon nuclear motions, especially upon vibrational frequencies, to consequently affect intra- and inter-molecular interactions [36] . As a result of deuterium’s larger mass, the vibrational amplitudes are smaller for deuterium, resulting in weaker non-covalent intermolecular interaction for deuterated P3HT than for the corresponding protonated P3HT. The absorption and PL of conjugated polymers follows the Frank-Condon transitions, which are coupled with their vibrational states as a result of electron–phonon coupling, and therefore the decreased absorption strength for the MD-P3HT indicates that deuteration of the thiophene ring is more effective than deuteration of the alkyl side chain in affecting non-covalent intermolecular interactions, such as π - π interaction. The less intense 0–1 PL peak at 665 nm of the deuterated P3HT ( Fig. 1c ) also indicates a weaker intermolecular interaction in deuterated blend films [37] . Owing to its low absorption coefficient, MD-P3HT/PCBM will absorb fewer photons, thereby generating fewer excitons and eventually resulting in a lower I sc . Although the electronic potential energy curves do not depend on the mass of the atoms in the molecule, the vibrational states are affected and can influence the mean lifetime of P3HT singlet excited states. As is clearly indicated from Raman spectroscopy, the vibrational modes of P3HT are changed significantly after deuteration, and this is consistent with the observed reduction in the excited state lifetime of deuterated P3HT. This reduction results from an increased non-radiative transition rate caused by the enhanced electron–phonon interaction resulting from deuteration [38] . We now turn our attention to the significantly reduced V oc observed in the SD-P3HT/PCBM blend, or more specifically, the drop in potential from 0.58 V for the protonated sample to 0.34 V for the deuterated sample. It should be noted that V oc for BHJ PV not only depends on the energy gap ( ΔE DA ) between the highest occupied molecular orbital (HOMO) energy of the donor and the lowest unoccupied molecular orbital (LUMO) energy of the acceptor, but on the ΔV loss related with interfacial charge transfer state and other recombination mechanisms [39] . Here, the observed V oc difference cannot be attributed to ΔE DA because the HOMO–LUMO level of SD-P3HT and MD-P3HT are similar to that of protonated P3HT (LUMO: −2.62 eV, HOMO: −4.84 eV) shown in Supplementary Fig. 5 . Based on the generalized Shockley equation under open circuit conditions, V oc is given as [40] , [41] , [42] , Where J 0 is the reverse saturation current, q is the elementary charge, kT is the thermal energy, n is the diode ideality factor, and J sc is the photocurrent. Figure 5a presents the J-V characteristics of protonated and deuterated P3HT/PCBM devices measured in darkness. Protonated P3HT and MD-P3HT shows similar J 0 , implying a similar V oc . However, J 0 for SD-P3HT/PCBM devices is almost two orders of magnitude higher than that of P3HT/PCBM, suggesting a smaller V oc. The parameters from the J-V characteristics fitted with the generalized Shockley equation are summarized in Supplementary Table 2 . We observe that the calculated V oc shows very good agreement with those obtained experimentally, and we make the argument that the small V oc of SD-P3HT OPV is well correlated with its large J 0. The physical origin of J 0 can be linked with the formation of a charge transfer state and bimolecular recombination at the interface. Recent studies show that V oc is proportional to the energy of the interfacial charge transfer state [34] , [43] . We note that the formation of an interfacial charge transfer state can be detected from sub-band absorption, photoluminescence, electroluminescence and magnetic field measurements [34] , [35] , [36] , [37] , [38] , [39] , [40] , [41] , [42] , [43] , [44] . The electroluminescence emission from the protonated and deuterated P3HT/PCBM blend ( Fig. 5b ) shows that MD-P3HT/PCBM has the same charge transfer emission without a clear spectral shift with protonated P3HT/PCBM, implying the same energy level for the charge transfer state. This result is consistent with the unchanged V oc after the main-chain deuteration. The absence of observable charge transfer emission for SD-P3HT/PCBM is either due to the low-energy charge transfer state, which may be shifted beyond our detector range, or due to enhanced non-radiative recombination caused by the side-chain deuteration. To further explore the side-chain deuteration effect on the reduced V oc , computational studies were carried out using a simple model system of an oligomer of 3-hexylthiophene and PCBM ( Supplementary Fig. 6 ). The rate of charge separation, K cs , and the rate of charge recombination, K cr , can be defined within a Marcus–Levich–Jortner rate equation [45] . A goal of polymer blend optimization is to extend carrier lifetimes sufficiently, increasing K cs , so that significant recombination losses, lower K cr , are pushed to higher carrier densities and therefore higher V oc . Deuteration of the P3HT hexyl side chain appears to effectively achieve the opposite: lower K cs and higher K cr . The root of this change is hypothesized to be due to a number of coupled processes resulting from changes in molecular properties brought about by isotopic substitution. First, the electronic coupling for charge separation, V cs , is lowered and the contribution from quantum vibrational modes, the internal and external reorganization energy is altered (due to different vibrational frequencies and density of states and a different polarizability of deuterium), as discussed below. Second, deuteration can reduce the presence of mixed phases of P3HT and PCBM due to the reduced miscibility. These changes originate from a shorter C-D bond length (hexyl side-chain deuteration causes a C-D bond length contraction of about 0.01 Å according to nuclear–electronic orbital calculations, see Supplementary Tables 3–5 ) and reduced electronic polarizability, which can lead to weaker intermolecular interactions. Also the reduced C-D dipole strength could result in a change in the work function of the cathode induced by interfacial dipoles, which would modify the internal electric field. All of these changes can affect V oc due to effectively modifying the energy required for formation of a charge transfer state. Isotope effects of H/D substitution on molecular polarizability, and refractive index have also been related to the changes in the zero-point energy of vibrations, and the polarizability isotope effect can be correlated with vibrationally averaged transition dipole moments. Based on density functional tight binding (DFTB) molecular dynamics simulations with dispersion corrections (see Methods for details) for the model P3HT/PCBM heterojunction, we computed several electronic structure properties that account for dynamical fluctuations that would be present in experimental measurements. In Supplementary Fig. 7 , the top panel shows the dynamically averaged HOMO–LUMO gap at different temperatures over a 10 ps trajectory. The root mean square of HOMO–LUMO gap increases with temperature because of increased spatial extent of the atomic motion. Overall, the results are consistent with experiment and indicate the HOMO–LUMO gap is effectively insensitive to side-chain deuteration. However, the time-averaged ΔE(HOMO)=E(HOMO)-E(HOMO-1) of the heterojunction at a given temperature is slightly more sensitive to deuteration. The general trend is that deuteration causes a small decrease in the electronic coupling and this difference increases with temperature. Examination of the electronic excited state shows that for the averaged structure of the SD-P3HT, the triplet state has larger electron density on the thiophene backbone than the protonated case shown in Supplementary Fig. 7c . While a larger model system is required to make more conclusive statements, these preliminary results provide an indication that exciton separation at the interface between SD-P3HT and PCBM will be less likely to occur. Finally, and most dramatically, deuteration affects the phonon dispersion curves and will alter electron–phonon coupling. An increase in electron–phonon coupling will reduce the FF and that is in accord with the results reported in Table 1 . It will also contribute to non-radiative electronic processes that decrease luminescence lifetime, in accord with Supplementary Fig. 2 . Overall, these combined effects-a decreased electronic coupling, charge transfer states and electron–phonon coupling-all contribute to the decrease in V oc and PCE. The neutron reflectivity curves for each blend film show that the vertical phase morphology of P3HT/PCBM and SD-P3HT/PCBM are essentially identical, but the composition profile of the MD-P3HT/PCBM film is clearly different from films of P3HT/PCBM and SD-P3HT/PCBM. Specifically, more PCBM is accumulated in the surface layer and the mid-layer adjacent to the surface layer in the MD-P3HT/PCBM film. It has been shown that the degree of PCBM diffusion in a P3HT matrix is closely related to the crystallinity of P3HT in that PCBM more easily passes through amorphous P3HT than crystalline P3HT [13] . In the present work, the crystallinity of P3HT and SD-P3HT were found to be comparable while that of MD-P3HT was significantly poorer. Consequently, this leads to the high degree of PCBM vertical diffusion to the air/film interface observed in MD-P3HT/PCBM, and as a result, we are able to conclude that selective deuteration of the side chain of P3HT does not change the phase separation morphology of SD-P3HT/PCBM, whereas deuteration of the polythiophene main-chain changes the vertical and lateral morphology in OPV. The realization that aromatic deuteration leads to a dramatic change in the phase separation in OPV blends greatly challenges the present paradigm. It underscores the need for a much more detailed understanding of the often neglected effects of deuterium substitution in neutron experiments. As a practical matter, deuteration of aromatic C-H in conducting polymers should be avoided for the design of deuterated materials for the neutron experiments. In summary, we have investigated how deuterium substitution in rr-P3HT, on both the thiophene backbone and on the alkyl side chains, affects the structure, morphology and optoelectronic properties of blend films used in OPV. A significant drop of nearly 50% in the PCE of P3HT/PCBM was noted after deuteration. Deuteration on the main-chain (MD-P3HT) and side-chain (SD-P3HT) were found to contribute differently to the photovoltaic characteristics. Specifically, MD-P3HT mainly reduces I sc without much change to V oc , while SD-P3HT exhibits a significant reduction of V oc (as large as 0.24 V) without a change in I sc . Structure and morphology studies demonstrated that MD-P3HT shows the lowest film crystallinity, the weakest intermolecular packing, and more random crystallites in P3HT/PCBM blends, all of which are responsible for the reduced I sc and OPV efficiency. The V oc loss in SD-P3HT/PCBM OPVs is attributed to a higher saturation dark current and the recombination of an interfacial charge transfer state. Moreover, neutron reflectivity measurements show that side-chain deuteration does not influence the vertical profile of P3HT/PCBM bulk films while main-chain deuteration does change the vertical and lateral morphology of P3HT/PCBM films. The origin of the changes in the optoelectronic properties of conducting polymers is attributed primarily to differences in the lengths of the C-D versus C-H covalent bonds, and secondarily to the changes in the physical properties of molecules that are a consequence of deuteration, such as changes in polarity, polarizability and molecular volume. Deuteration of the thiophene ring of P3HT generally is more effective than deuteration of the alkyl side chain in affecting the non-covalent intermolecular interactions, resulting in different optoelectronic properties. Our experimental and theoretical results of the isotopic effects of deuterium substitution on the structure, morphology and optoelectronic responses of model P3HT/PCBM systems indicates that isotope effects have significant impact on the optoelectronic properties of conducting polymers and the crucial photovoltaic processes in OPV devices such as charge transport and V oc . Such effects require continued investigation and practical consideration when planning experiments or interpreting the results of experiments involving the use of deuterium labelled compounds, especially for the neutron scattering/reflectometry experiments. Materials Synthesis The synthesis of rr-P3HT is referred to previous publication [46] . The synthetic route of deuterated P3HT was shown in Supplementary Fig. 1 . Dry THF was used as the solvent through the synthesis. Side-chain-deuterated P3HT was obtained from adopted literature procedures by reacting of 3-bromothiophene and 1-bromohexane-d13 under refluxing [29] . 2,5-Dibromo-3-hexylthiophene-d13 was polymerized using the Kumada catalyst transfer polymerization method. The polymer was collected and purified by Soxhlet extraction with methanol, hexanes and chloroform sequentially. The chloroform fraction was precipitated in large excess methanol and freezed dry over benzene for 24 h. The overall yield was around 25%. The synthesis of main-chain-deuterated P3HT was carried out similarly and the overall yield of the polymer was about 19%. The polymers were characterized with 1 H NMR (500 MHz) and 13 C NMR (125 MHz) in CDCl 3 . Relative MW (to PS standards) of the polymers were obtained by GPC in THF (1 ml min −1 ). Element analysis: calcd. C 71.86; H/D, 8.98; S , 19.16 (main-chain deuterated), C 67.03; H/D, 15.08; S , 17.88 (side-chain-deuterated), Found: C , 68.51; H , 8.01; S , 17.95 (main-chain deuterated); C , 64.77; H/D, 13.46; S , 16.13 (side-chain deuterated). The off-marked EA might be due to chain ends (Br), but the purities of these polymers are comparable. The regioregularity (HT–HT coupling) is better than 98.3% by NMR. Thin film characterization UV–vis absorption spectra were recorded using a Varian Cary UV–vis-NIR spectrophotometer. PPL measurements were made using a Jobin–Yvon Fluoromax-2 spectrometer at the excitation wavelength of 550 nm. Raman spectra of P3HT isotopes were recorded by a Renishaw 1000 confocal microRaman spectrometer with an excitation wavelength of 633 nm. Atomic force microscope images were acquired with a Bruker Dimension Icon operating in a tapping mode. Transmission electron microscopy (TEM) investigations were performed using a Zeiss Libra 120 with an in-column energy filter. Selected area electron diffraction patterns were calibrated against Au (111) standards (0.2335, nm). GISAXS and GIWAXS measurements were performed at the 8ID-E beam-line at the advanced photon source (APS), Argonne National Laboratory using X-rays with a wavelength of λ =1.6868 Å and a 2-D PILATUS 1M-F detector that was situated at 208.7 mm from samples. NR measurements were performed on the Liquids Reflectometer (Beam line 4B) at the Spallation Neutron Source (SNS), Oak Ridge National Laboratory (ORNL). The lifetimes of the singlet states of P3HT isotopes and P3HT/PCBM blends were measured using a picosecond time-correlated single-photon-counting (TCSPC) setup, which has been described in detail previously [47] . Device fabrication and measurement Synthesized P3HT isotopes were blended with PCBM (1:0.7 wt%) and subsequently dissolved in 1,2-dichlorobenzene at a concentration of 20 mg ml −1 . The P3HT/PCBM blend solution was heated on hotplate at 60 °C overnight before device fabrication. Indium tin oxide (ITO) substrates were sequentially ultrasonically agitated in detergent, DI water, acetone and isopropyl alcohol. The cleaned ITO substrates were treated with UV Ozone for 20 min. PEDOT:PSS was spin coated onto the ITO substrates with a film thickness of 40 nm. After baking the PEDOT films in air at 120 °C for 1 h, The P3HT:PCBM blend solution was then spin coated on top of PEDOT:PSS layer with a film thickness of 80 nm. The films were thermal annealed at 140 °C for 20 min in a vacuum oven. Finally, the fabrication of bulk heterojunction OPV devices were then completed by thermal evaporation of 20-nm Ca and 70-nm Al films through a shadow mask. More than 70 OPV devices were fabricated and tested, and showed good reproducibility. Organic field-effect transistors were fabricated in the bottom-gate bottom-contact configurations. Heavily doped n -type Si substrates served as the gate electrodes, and a 100-nm thick thermally grown silicon dioxide overlayer were used as the dielectric layer. The source and drain electrodes were patterned using standard photolithography methods followed by sequential e-beam deposition of 10 nm of Ti and 60-nm of Au. P3HT isotopes films were spin-coated from 10 mg ml −1 from trichlorobenzene solution and annealed at a vacuum oven at 130 °C for 1 h. Current voltage characterization of OPVs were conducted using a Keithley 4200 semiconductor parameter analyser under AM 1.5 conditions (100 mW cm −2 ). The electrical measurements of the OFET were carried out in air with a Keithley 4200 semiconductor parameter analyser and a probe station. Density functional theory calculations To study the structural, dynamical and electronic response of side chain deuteration, we employed self-consistent charge density functional tight-binding (SCC-DFTB) simulations [48] , [49] , [50] . Structural optimization of a model PCBM/P3HT heterojunction, represented here as a single molecule for the donor and acceptor (see Supplementary Fig. 7 ), was performed with the inclusion of an empirical dispersion term [49] to account for weak non-covalent interactions. To analyse the effects of P3HT side-chain deuteration a set of NVT (Nose–Hoover thermostat) molecular dynamics simulations for the model PCBM:P3HT heterojunction were performed. To mimic the bulk heterojunction, the PCBM and backbone of P3HT were constrained while the hexyl side chains were allowed to be fully dynamic. Each DFTB trajectory used a 1 fs time step and was run for a total 10 ps. The simulations were performed at various constant temperatures ranging from 5 to 50 K. The molecular geometries were recorded during the simulations every 10 fs (1,000 snapshots over the 10 ps trajectory). These results were then averaged to account for the dynamical fluctuations at each temperature. Fluorescence lifetime measurements The singlet excited state lifetimes of P3HT isotopes and P3HT:PCBM blends were measured by a picosecond TCSPC setup, which was described in detail previously [47] , so only a brief account will be given here. The detection system includes an actively quenched single-photon avalanche photodiode (PDM 50CT module, Micro Photon Devices) and a TCSPC module (PicoHarp 300, PicoQuant). The light source was an optical parametric amplifier pumped by a 250 kHz Ti:Sapphire regenerative amplifier. Excitation was at 550 nm with typically 50 fs (full width at half maximum, FWHM) pulse duration and<0.1 nJ pulse energy. Fluorescence emission was selected by using a 10 nm (FWHM) bandpass filter centred at 660 nm, which was chosen according to the peak wavelength of the fluorescence emission spectra. The instrument response function (IRF) showed a FWHM of~40 ps as recorded at the excitation wavelength using a dilute water suspension of coffee creamer. A 4.0-ps channel time was chosen and the polarization of the excitation beam was set to the magic angle (54.7°) with respect to an emission linear polarizer. Measurements at higher pulse energies were also performed to verify that the decay kinetics is independent of excitation intensity. Data were also taken for different sample positions to ensure reproducibility. Quantitative analysis of the time-resolved fluorescence data were performed by employing a least squares deconvolution fitting algorithm with explicit consideration of the finite instrument response function (FluoFit, PicoQuant) and a reduced chi square (χ 2 ) value is used to judge the quality of each fit. Grazing incidence and wide-angle and small-angle X-ray scattering GIWAXS and GISAXS measurements were performed using Beamline 8ID-E at the Advanced Photon Source (APS), Argonne National Laboratory. Scattering intensities are expressed as a function of the scattering vector, q =4 π / λ sin θ , where θ is the half scattering angle and λ =1.6868 Å is the wavelength of the incident radiation. The d -spacing of a peak is expressed by 2 π / q . A two-dimensional area detector was used to collect the scattering images and was situated at 200.4 or 158.6 mm from the sample for GIWAXS measurements. The films were illuminated by X-rays at 7.35 keV at an incidence angle of about 0.2°. Information about in-plane nanoscale phase structure formed in thin film can be obtained by GISAXS. Supplementary Fig. 3a–c shows 2D GISAXS patterns of P3HT/PCBM, MD-P3HT/PCBM and SD-P3HT/PCBM films. Also, the in-plane 1D GISAXS profiles were deduced from the 2D patterns and depicted in Supplementary Fig 3d–f . In order to obtain more detailed information about the high electron density PCBM phase domains present in low electron density P3HT matrices, the extracted in-plane GISAXS profiles were fit by combining Guinier-Porod model [51] and polydisperse sphere model with Schulz size distribution [52] as shown in Supplementary Fig. 3d–f . As seen from the fit results, the combined model gave rise to a goodness of fits. In the model fits, Guinier-Porod and polydisperse sphere model account for PCBM phase domains with largely two different sizes, that is, Guinier-Porod model for larger domains (low- q y region) and polysphere model for smaller phase domains (high- q y region). The fit parameters used to fit the GISAXS curves are tabulated in Supplementary Table 1 . NR measurements Neutron reflectivity measurements were conducted at the SNS in ORNL using the Liquids Reflectometer (BL-4B). Specular reflectivity data were collected in a continuous wavelength band (2.5 Å< λ <6.0 Å) and eight different incident angles, α ; α ≈0.17°, 0.27°, 0.34°, 0.48°, 0.62°, 1.11° and 2.01° and 3.62° were used. From these instrument settings, we have acquired reflectivity data covering a wide wave vector transfer ( q =4 π sin θ / λ ) range of 0.007 Å –1 < q <0.278 Å –1 . To fit the data, the initial thicknesses measured using ellipsometry were considered and thicknesses, SLD and interfacial widths were adjusted to achieve best fit of the model with the NR data. The NR model fits were based on the Parratt formalism and the interfacial structure is modelled using the distribution proposed by Nevot and Croce. Also, the volume fraction of PCBM as a function of z , F PCBM ( z ), is calculated from the SLD profiles and equations (1) and (2). Using the fitting parameters i.e. , β i , i,i+1 and z i,i+1 that were used to fit the NR data in Fig. 6b , F PCBM ( z ) can be given as, where the weight fraction of PCBM in i th layer, F PCBM ,i is directly calculated from the relation, as, where w PCBM,i (1- w P3HT,i ) is the weight fraction of PCBM in the i th layer. Theoretical investigation of isotope effects in 3-hexylthiophenes Computational study of the effects of deuteration for a single monomer of 3-hexylthiophene (3HT, Supplementary Fig. 6 ) were also performed using the Nuclear–Electronic Orbital (NEO) method [53] . In the NEO method, nuclear quantum effects are incorporated into an electronic structure calculation by treating specified nuclei quantum mechanically. Electronic and nuclear orbitals are expressed as linear combination of Gaussian basis functions, and the energy is minimized variationally with respect to all molecular orbitals, as well as the centres of the nuclear basis functions. All calculations were performed using the NEO implementation included in the GAMESS electronic structure code [54] . Calculations were performed at the Hartree–Fock level using the 6-31G** basis for the electronic wave function and a double-zeta basis composed of two s-type Gaussian functions for each quantum mechanical nucleus for the nuclear wave function. First, calculations using the standard DZSNB NEO nuclear basis were performed, successively the Gaussian exponents of the nuclear basis were optimized in order to reproduce the experimental vibrational frequencies of P3HT in both pure and deuterated forms. In the NEO calculations, all the hydrogen atoms of the hexyl chain were treated quantum mechanically, for a total of 13 quantum nuclei, while the hydrogens attached to the thiophene ring were not included in the nuclear wave function. The high spin configuration, where all nuclear spins are parallel, was chosen for the nuclear wave function. To simulate deuteration in the NEO calculation, the mass of the quantum nuclei was changed from 1,836 a.u. (hydrogen) to 3,672 a.u. (deuterium). How to cite this article : Shao, M. et al. The isotopic effects of deuteration on the optoelectronic properties of conducting polymers. Nat. Commun. 5:3180 doi: 10.1038/ncomms4180 (2014).